Genomic landscape and genetic heterogeneity in gastric adenocarcinoma revealed by whole-genome sequencing Gastric cancer (GC) is the second most common cause of cancer-related deaths. It is known to be a heterogeneous disease with several molecular and histological subtypes. Here we perform whole-genome sequencing of 49 GCs with diffuse ( N =31) and intestinal ( N =18) histological subtypes and identify three mutational signatures, impacting TpT, CpG and TpCp[A/T] nucleotides. The diffuse-type GCs show significantly lower clonality and smaller numbers of somatic and structural variants compared with intestinal subtype. We further divide the diffuse subtype into one with infrequent genetic changes/low clonality and another with relatively higher clonality and mutations impacting TpT dinucleotide. Notably, we discover frequent and exclusive mutations in Ephrins and SLIT/ROBO signalling pathway genes. Overall, this study delivers new insights into the mutational heterogeneity underlying distinct histologic subtypes of GC that could have important implications for future research in the diagnosis and treatment of GC. Gastric cancer (GC) is a heterogeneous disease with two distinct morphologic subtypes—intestinal and diffuse—showing variable environmental aetiologies, clinical manifestation and genetic background [1] . The diffuse-type GC is more often seen in female and young individuals, while the intestinal-type adenocarcinoma is more often associated with intestinal metaplasia and Helicobacter pylori infection [2] . Previous whole-exome sequencing studies analysed 22 (3 diffuse-type) and 15 (2 diffuse-type) gastric adenocarcinomas and showed frequent inactivating mutations in cell adhesion and chromatin remodelling genes in addition to TP53 mutations [3] , [4] . However, the complete spectrum of genetic changes in GCs remains largely undefined. Furthermore, stroma-dominant growth pattern and subsequent small cancer cell population within tumour has so far restricted application of large-scale next-generation sequencing studies on diffuse-type GC [3] . Recent comprehensive molecular characterization of GC proposed a molecular classification dividing GC into four subtypes [5] , and large-scale genomic studies reported gain-of-function mutations of RHOA in 0–25.3% of diffuse-type GCs [5] , [6] , [7] , [8] . However, some of those were performed with relatively low coverages (~6.19X (ref. 5 ) and 32X (ref. 7 )). Human cancers result from a complex series of genetic alterations, resulting in heterogeneous disease states. Dissecting this heterogeneity is critical for understanding underlying mechanisms and providing opportunities for therapeutics matching the complexity [9] . However, intratumoral genetic heterogeneity during gastric tumour progression has not been comprehensively investigated so far. To improve understanding of the genomic basis of diffuse-type GC and identify the underlying genetic heterogeneity, we perform whole-genome sequencing (WGS) of tumour and matched peripheral blood samples from 49 patients with advanced stage (stage IV, 19; stage III, 29; stage II, 1), 31 diffuse and 18 intestinal subtype, microsatellite-stable (MSS) GCs ( Supplementary Data 1 ). Deep sequencing (>100X coverage) combined with high tumour cell content enables us to identify mutational heterogeneity in GCs and genetic alterations underlying diffuse subtype of gastric adenocarcinoma. Overview of the GC genome DNA from both tumour and peripheral blood mononuclear cells (PBMC) was sequenced using unchained combinatorial probe anchor ligation chemistry on arrays of self-assembling DNA nanoballs [10] . The median genome coverage was 105X for the tumours and 91X for the control PBMC samples. The median of fully called genome fractions (that is, percentage of reference bases for which all alleles were called) was 97.3% for tumours and 96.8% for PBMC samples, respectively. The percentage of the genome covered at 10X or more was 98.9% for the tumour and 98.4% for the control. The number of somatic variants per tumour patient genome varied greatly (median, 9,036; range, 172–38,328) ( Fig. 1a and Supplementary Data 2 ). In the coding regions, the median number of mutations per sample was 94 (range: 2–321). The median mutation rate for the coding regions (~2.36 per Mb) was lower than the rate for both intronic (~2.56 per Mb, P =1.2E−4) and intergenic (~3.3 per Mb, P =3.1E−6) regions. The percent of somatic single-nucleotide changes associated with C>A, C>G, C>T, T>A, T>C, T>G was distributed as 15.12, 6.20, 26.87, 10.09, 20.12 and 21.60%, respectively, across the whole genome and 13.44, 6.34, 51.78, 6.22, 13.06 and 9.17% across the coding regions ( Supplementary Data 2 ). 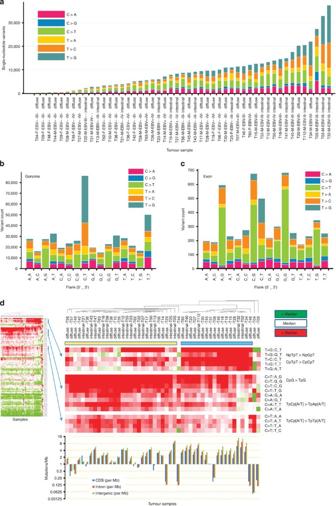Figure 1: Mutational load and mutational signatures in 49 gastric cancers. (a) Mutational load: stacked bar plot of the single-nucleotide variant (SNV) count (y-axis) and nucleotide change with the changes indicated by the following colours: C>A (magenta), C>G (blue), C>T (green), T>A (yellow), T>C (orange) and T>G (grey). The tumour samples (x-axis) are ordered by the number of nucleotide variants, and each patient sample identifier is annotated with sex (M/F), EBV status (+: positive, −: negative), stage and Lauren histological classification (intestinal or diffuse). (b,c) Stacked bar plot of the SNV count and nucleotide changes in different trinucleotide sequence contexts for whole-genome (b) and -exome (c) regions. The flanking base pairs are arranged in the 5′ to 3′ direction in 16 categories (x-axis), for a total of 96 possible flanking nucleotide and SNV combinations. (d) Hierarchical cluster of 96 possible combinations of the flanking sequences and SNVs. Thex-axis: tumour sample;y-axis: the trinucleotide context and corresponding SNVs. The SNV counts were converted to fractions to avoid co-clustering of samples with high single-nucleotide variant counts. The tumour samples largely cluster into two groups as marked by the yellow and blue bars. Three mutational patterns emerge: (1) TpT nucleotide, NpTpT>NpGpT and TpTpT>TpCpT (mostly impacting a subgroup of the diffuse tumour subtype, with a high mutational load); (2) CpG island-related regions, CpG>TpG and (3) TpCp[A/T]>TpTp[A/T] and TpCp[A/T]>TpAp[A/T], representing APOBEC mutational patterns related to TCW motifs (W=A/T). Samples with a CpG mutational have a reduced presence of the TpT-related pattern. The mutational load in the exonic, intronic and intergenic regions is provided in the lower panel, with samples arranged in the same order as the hierarchical cluster above. Samples with the TpT mutational pattern (highlighted by a blue bar) tended to occur largely in a subset of diffuse-type GCs and showed a much higher mutation rate in intergenic and intronic regions than in coding regions compared with the remaining samples. Figure 1: Mutational load and mutational signatures in 49 gastric cancers. ( a ) Mutational load: stacked bar plot of the single-nucleotide variant (SNV) count (y-axis) and nucleotide change with the changes indicated by the following colours: C>A (magenta), C>G (blue), C>T (green), T>A (yellow), T>C (orange) and T>G (grey). The tumour samples ( x -axis) are ordered by the number of nucleotide variants, and each patient sample identifier is annotated with sex (M/F), EBV status (+: positive, −: negative), stage and Lauren histological classification (intestinal or diffuse). ( b , c ) Stacked bar plot of the SNV count and nucleotide changes in different trinucleotide sequence contexts for whole-genome ( b ) and -exome ( c ) regions. The flanking base pairs are arranged in the 5′ to 3′ direction in 16 categories ( x -axis), for a total of 96 possible flanking nucleotide and SNV combinations. ( d ) Hierarchical cluster of 96 possible combinations of the flanking sequences and SNVs. The x -axis: tumour sample; y -axis: the trinucleotide context and corresponding SNVs. The SNV counts were converted to fractions to avoid co-clustering of samples with high single-nucleotide variant counts. The tumour samples largely cluster into two groups as marked by the yellow and blue bars. Three mutational patterns emerge: (1) TpT nucleotide, NpTpT>NpGpT and TpTpT>TpCpT (mostly impacting a subgroup of the diffuse tumour subtype, with a high mutational load); (2) CpG island-related regions, CpG>TpG and (3) TpCp[A/T]>TpTp[A/T] and TpCp[A/T]>TpAp[A/T], representing APOBEC mutational patterns related to TCW motifs (W=A/T). Samples with a CpG mutational have a reduced presence of the TpT-related pattern. The mutational load in the exonic, intronic and intergenic regions is provided in the lower panel, with samples arranged in the same order as the hierarchical cluster above. Samples with the TpT mutational pattern (highlighted by a blue bar) tended to occur largely in a subset of diffuse-type GCs and showed a much higher mutation rate in intergenic and intronic regions than in coding regions compared with the remaining samples. Full size image We observed tens of mutations in coding regions per patient sample; the majority appears to be passenger rather than driver mutations. Recent work has shown that a very large proportion of mutations may have appeared before tumour initiation and that the number of somatic mutations in tumours of self-renewing tissues are positively correlated with the age of the patient at diagnosis [11] . In support of that, we see a trend that younger patients below the age of 55 ( N =15/49) in our cohort tend to have much smaller number of mutations (2.16 vs 3.88 mutations per Mb; P =0.018). To study the mutational processes, we analysed the trinucleotide sequence context of the variants in the coding and non-coding regions ( Fig. 1b,c , Supplementary Data 3 ). Exonic regions exhibited a very high frequency of NpCpG>NpTpG ( N =A/T/G/C) mutations, whereas NpTpT>NpGpT changes were more common in the entire genome. We looked at the mutational signatures using the relative frequency of each of the 96 possible trinucleotide combinations using hierarchical clustering. Hierarchical cluster revealed three patterns: (a) TpT dinucleotide (unknown mechanism, observed in oesophageal cancer) [13] , (b) CpG (CpG island-related regions) and (c) TpCp[A/T] ( APOBEC mutational pattern impacting TCW motif, where W=A/T) [14] . Samples with the TpT mutational pattern ( N =18/49) tended to occur largely in a subset ( N =14/18) of diffuse-type GCs, with tubular cell morphology ( N =14/18) and showed a much higher mutation rate in intergenic ( P =0.006) and intronic ( P =0.012) regions than in coding regions ( P =0.096) compared with the remaining samples ( Fig. 1d ). Only four of 18 intestinal-type GCs had this mutational signature. Moreover, GCs with a CpG mutational signature had a reduced presence of the TpT-related pattern. In total, there were 4,528 exonic somatic mutations, consisting of 3,328 non-synonymous and 1,200 synonymous mutations; these mutations spanned 2,553 genes, with 384 being mutated in at least two tumours ( Supplementary Data 4 ). The median number of non-synonymous mutations detected per patient was 68 (range: 1–248), which was consistent with two previous exome-sequencing studies on GC [3] , [4] . Moreover, the median number of mutations per megabases (Mb) in the coding regions was similar to that reported for other cancers of the gastrointestinal tract, although our upper range was significantly lower owing to the lack of hypermutated tumours [15] . The diffuse-type GCs tend to have lower number of variations compared with intestinal-type GCs (2.41 per Mb vs 4.97 per Mb; P =0.009). We performed targeted resequencing using the selected 384 recurrent gene set identified from the WGS data (See Methods and Supplementary Data 5 ) and validated ~90% of the somatic mutations. We identify significantly mutated genes [16] ( Supplementary Data 6 ), reaffirming known mutations in GC ( TP53 , ARID1A , TGFBR2 and CDH1 ) [3] , [4] , and uncovered novel mutated genes including SYNE1 ( N =10, 20%) and TMPRS S2 ( N =3, 6%). Mutations of SYNE1 have been frequently reported in oesophageal adenocarcinoma and glioblastoma [13] , [17] . We also observed TGFBR2 mutations, but none of them were inactivating frameshift or nonsense mutations frequently observed in microsatellite instability (MSI)-high GC [18] , [19] , but, instead, we observed its potential activation in MSS GC and warrants further investigation of its role in MSS tumours. We found RHOA mutations (50G>A, p.Gly17Glu and 169T>G, p.Leu57Val) in 2 out of 31 (6.5%) diffuse-type GCs. In addition, we checked for known deleterious germline variants with known predisposition to GC. Two patients (T28 and T62) with diffuse-type GC showed CDH1 germline variant 2494G>A (heterozygous in both PBMC and tumour, corresponds to p.Val832Met), which has previously been described and characterized as pathogenic [20] , [21] . This is a known variant implicated in hereditary diffuse-type GC. Two patients (T10 and T18) with diffuse-type GC had TP53 germline variant 91G>A (heterozygous in both PBMC and tumour, corresponds to p. Val31Ile), which is previously reported in GC associated with Li Fraumeni syndrome [22] . Sample T10 had no other somatic mutation in TP53 ; however, T18 harboured somatic nonsense mutation of TP53 . In those patients, review of medical records showed no family history of GC, suggesting that this variant may not have a high penetrance. Structural variations, such as tandem duplications, deletions and fusions, were frequently present across the genomes of the 49 GCs ( Fig. 2a , Supplementary Data 7 ). Intestinal-type GC showed significantly frequent structural variations compared with diffuse-type GC ( P ≪ 0.0004). Some GCs showed a very large number of tandem duplication events (for example, T02 and T30), while others (for example, T05 and T40) showed large genomic regions with deletions (large regions with loss of heterozygosity). 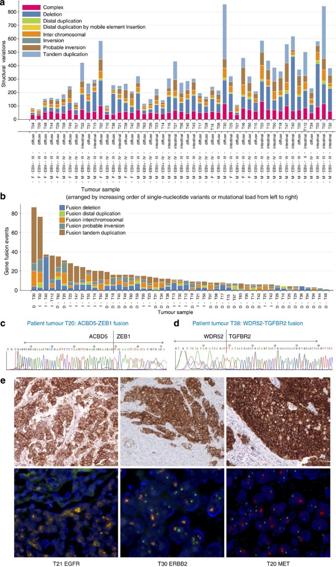Figure 2: Types of structural variations in gastric cancer. (a) Stacked bar plot of the structural variations. The tumour samples (x-axis) are ordered by the number of nucleotide variants and Lauren histologic classification (intestinal or diffuse). They-axis shows the number of somatic structural events, with eight types of events shown in different colours as reported by the Complete Genomics pipeline and described in theSupplementary Methods. (b–d) Stacked bar plot of gene fusion events (subset of structural variations). Thex-axis shows the tumour sample with intestinal and diffuse types labelled by ‘I’ and ‘D’, respectively, and they-axis shows the total number of fusion events observed. The fusions ofACBD5-ZEB1(c) andWDR52-TGFBR2(d) are validated by RT-PCR and sequencing. (e) DNA copy-number gains ofEGFR,ERBB2andMETconfirmed by immunohistochemical staining (upper panels) and fluorescencein situhybridization (lower panels). Figure 2: Types of structural variations in gastric cancer. ( a ) Stacked bar plot of the structural variations. The tumour samples ( x -axis) are ordered by the number of nucleotide variants and Lauren histologic classification (intestinal or diffuse). The y -axis shows the number of somatic structural events, with eight types of events shown in different colours as reported by the Complete Genomics pipeline and described in the Supplementary Methods . ( b – d ) Stacked bar plot of gene fusion events (subset of structural variations). The x -axis shows the tumour sample with intestinal and diffuse types labelled by ‘I’ and ‘D’, respectively, and the y -axis shows the total number of fusion events observed. The fusions of ACBD5-ZEB1 ( c ) and WDR52-TGFBR2 ( d ) are validated by RT-PCR and sequencing. ( e ) DNA copy-number gains of EGFR , ERBB2 and MET confirmed by immunohistochemical staining (upper panels) and fluorescence in situ hybridization (lower panels). Full size image We focused on gene fusion by examining putative partners for strand, orientation consistency as well as being in-frame. We observed that gene fusion events varied widely between tumours ( Fig. 2b , Supplementary Data 8 ). For example, tumours T02 and T30 showed 76 and 86 gene fusion events with resolved breakpoints, respectively, while tumours T48 and T44 only showed two and one resolved fusions, respectively. We narrowed our focus to 12 fusion gene pairs (found in 25 GC cases) based on recurrent and known cancer-related genes and confirmed ACBD5-ZEB1 (T07) , WDR52-TGFBR2 (T38), SOBP-MET (T07) and LACE1-MET (T20) fusions by RT-PCR and Sanger sequencing (See Methods and Fig. 2c,d ). In sample T20 with MET fusion, we observed MET amplification and mRNA and protein overexpression of MET . So, in this case, it is uncertain whether overexpression of MET mRNA and proteins is caused by fusion events or gene amplification. In sample T07, there was no overexpression of MET proteins by immunohistochemistry. Fusion genes other than WDR52-TGFBR2 may have been byproducts of tandem duplications as ZEB1 and MET were genetically amplified. It can’t be ascertained whether the fusion helped drive a higher expression of the genomic amplification, except to say that the fusion was in-frame. The fusion product of ACDB5-ZEB1 likely results in the overexpression of ZEB1, which is a transcriptional repressor of CDH1 , a key gene involved in gastric carcinogenesis. The inactivation of TGFBR2 has been implicated in MSI-high GC [19] ; however, we observed its potential activation in the present study and its functional roles in MSS tumours need to be elucidated. Recent TCGA results on GC reported fusion in CLDN18 with ARHGAP6 or ARHGAP26 , and this fusion events occurred mutually exclusive with RHOA mutation [5] . In our WGS results, we do not have any fusions on ARHGAP6 or ARHGAP26 or CLDN18 . We have a potential fusion by deletion of RHOA-GPX1 , but, on closer look, what is left is the upper and downstream of RHOA with no product. Another case is a potential fusion of RBM6 - RHOA by probable inversion with possible out-of-frame of partial RBM6 with full RHOA , which has no significant biological effect. We utilized WGS data from both gene-level structural variations and relative coverage (Methods and Supplementary Data 9 ) to estimate and summarize the copy-number alterations for each sample and the data set, respectively. The recurrent gains were observed in 7p12 ( EGFR , N =5), 19q12 ( CCNE1 , N =5), 18q11 (G ATA6 , N =5), 17q12–q21 ( ERBB2 , N =8), 7q21 ( CDK6 , N =3), 12p12 ( KRAS , N =3), MET ( N =2), 8q24 ( MYC , N =3) and 10q26 ( FGFR2 , N =2) and most of these loci have been reported in GCs [23] . As reported earlier, the gains in receptor tyrosine kinases and downstream effectors such as KRAS were largely mutually exclusive except for GATA6 , which co-occurred with other alterations in 80% of cases. For gene deletions, fragile sites such as FHIT ( N =29) and WWOX ( N =10) frequently showed aberrations, whereas CDH1 ( N =4), STK3 ( N =4), CTNNA1 ( N =3), PARD3 ( N =3) and RB1 ( N =1) were less frequently deleted. We confirmed EGFR , MET and ERBB2 copy-number alteration by using fluorescent in situ hybridization (FISH) and its consequent overexpression by immunohistochemistry ( Fig. 2e ). In almost all cases, gene copy-number gains led to a corresponding protein overexpression ( Supplementary Data 10 ). Clonal Heterogeneity of GC To assess clonal heterogeneity of GC, we segregated the observed somatic variations into clonal (that is, present in almost all cancer cells), subclonal (that is, present in a subset of cancer cells) and subclonal-del (heterogeneity in mutation: mutation in one copy of gene along with loss of other gene copy in subset of cancer cells and homozygous loss in remaining cancer cells). We first estimated the tumour purity and ploidy using ASCAT [24] of all samples and used that to further infer average copy number of the mutant allele (mCN) and tumour cell mutant-allelic fraction (tMAF). Using this, we segregated each mutation into clonal, subclonal or subclonal-del. The information over all genes was then used to estimate the tumour clonality of all samples (See methods for detailed explanation). We arranged the tumours in the order of increasing clonality and plotted the total variants ( Fig. 3a ), percentage of variants that are clonal and ploidy of tumour cells ( Fig. 3b ). We observed that the intestinal-type GC showed significantly higher ploidy ( P =0.019) and clonality ( P =0.009) than the diffuse type. To exclude the possibility of tumour cell contents affecting the estimated clonality or ploidy, tumour cells populations in two histologic subtypes of GC were compared. However, there was no significant difference ( P =0.32) between two subtypes, suggesting that purity did not confound estimated clonality or ploidy. Also, we did not observe any relationship between clonality and the TpT mutational signature. 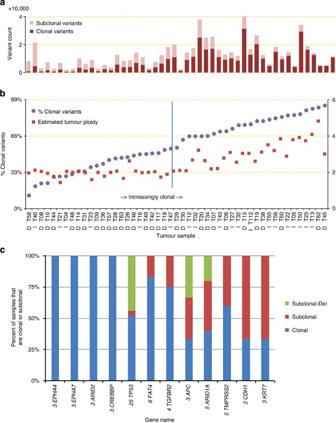Figure 3: Clonal analysis of gastric cancers. (a) Stack plot of SNVs segregated into clonal and subclonal variants. Thex-axis: tumour sample;y-axis: number of somatic variants in the 10,000s. (b) Plot of clonality and ploidy. The samples are sorted in ascending order of estimated clonality. The samples are also annotated according to Lauren classification (I: intestinal and D: diffuse subtype GC). The diffuse histological subtype samples tend to be diploid and show a lower percentage of clonal variants and lower number of variants. By contrast, the intestinal subtype samples show polyploidy and tend to be more clonal. (c) Clonal and subclonal mutation percentage counts across all tumours for selected recurrent mutated (non-silent) genes in at least three tumours. Thex-axis is labelled with the sample count and gene name, and they-axis is the tallied percentage for each classification. Potential existence of cells with homozygous deletion in some cells along with cells harbouring mutation in one gene copy with loss of other copy in the same tumour sample was labelled as subclonal-del. Figure 3: Clonal analysis of gastric cancers. ( a ) Stack plot of SNVs segregated into clonal and subclonal variants. The x -axis: tumour sample; y -axis: number of somatic variants in the 10,000s. ( b ) Plot of clonality and ploidy. The samples are sorted in ascending order of estimated clonality. The samples are also annotated according to Lauren classification (I: intestinal and D: diffuse subtype GC). The diffuse histological subtype samples tend to be diploid and show a lower percentage of clonal variants and lower number of variants. By contrast, the intestinal subtype samples show polyploidy and tend to be more clonal. ( c ) Clonal and subclonal mutation percentage counts across all tumours for selected recurrent mutated (non-silent) genes in at least three tumours. The x -axis is labelled with the sample count and gene name, and the y -axis is the tallied percentage for each classification. Potential existence of cells with homozygous deletion in some cells along with cells harbouring mutation in one gene copy with loss of other copy in the same tumour sample was labelled as subclonal-del. Full size image To segregate the initial vs late-acquired mutations, we studied the clonality of recurrently mutated genes (non-silent variants) present in at least 3 out of 49 tumours. This analysis revealed that ARID2, EPHA7 and EPHA4 genes were involved in GC initiation, whereas mutations of FAT4, TGFBR2, APC, ARID1A, CDH1 and PIK3CA [25] were present in a subset of cancer cells, suggesting later involvement in tumour progression ( Fig. 3c ) [25] . Some of the genes were tumour suppressors with two apparent modes of gene loss coexisting in the tumours, that is, mutation with one copy loss in some cells and a homozygous deletion of gene in other cells, leading to a functional loss in more than one way ( Supplementary Data 11 ). TP53 , the most frequently mutated gene in GC, was clonal in 52% of GC and subclonal-del (some cells harbour a homozygous deletion and others have a copy loss and mutation each) in 44% of cases, suggesting that intratumoral heterogeneity exists in TP53 -inactivation mechanism. Integrative plot and pathway analysis of recurrent mutations An integrative plot of the genetic aberrations, clinical covariates, clonality and mutational signatures ( Fig. 4a ) revealed predominantly mutually exclusive copy-number gains in receptor tyrosine kinases as previously described [26] . Most of these gains were observed in a TP53 -mutant background [27] . A subset of the diffuse-type GCs ( N =13/31, Fig. 4a , far right blue box on axis) was mostly diploid and showed very few genetic alterations and a low mutational load (‘genetically quiet’). We observed mutations in CDH1 , CTNNA1 or PIK3CA genes in ‘genetically quiet’ diffuse-type GCs. Germline mutations of CTNNA1 (ref. 28 ) or CDH1 (ref. 29 ) genes have been reported in hereditary diffuseGCs, and frequent PIK3CA mutations were observed in diffuse-type sporadic GCs [7] . On the basis of recent whole-genome and sequencing results on diffuse-type GCs, high mutation rates of CDH1 , CTNNA1 or PIK3CA may specifically contribute to the carcinogenesis of diffuse-type GCs. In contrast, the diffuse-type GCs with TpT mutational signature were irrespective of the genetically quiet tumours, suggesting two different mutational mechanisms operating within diffuse-type GC. 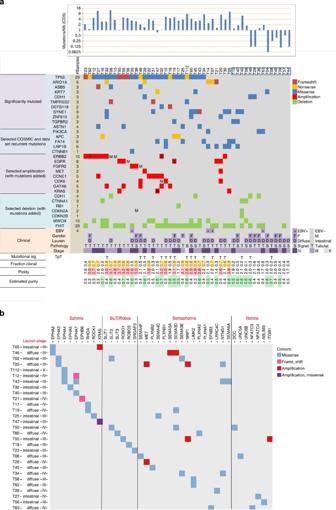Figure 4: Landscape of key genetic alterations in gastric cancers. (a) The patient samples are shown on thex-axis. On they-axis (top to bottom panel), the coding region mutation rate, top 12 significantly mutated genes, selected COSMIC and recurrent mutated genes, recurrent copy-number alterations (gains and deletions), clinical information, presence of TpT mutational signature, clonality, ploidy and purity are provided. The number of patients with an observed alteration type or types in given in the second column in the lower panel marked as ‘#Samples’. Different mutation and genomic alteration types are shown in different colours. Additional information is added as follows. Genes in the copy-number alterations have been marked with ‘M’ if they carried a non-synonymous mutation; ‘X’ did not show overexpression of protein by immunohistochemistry; ‘?’ for ambiguous results. The rows related to clonality, ploidy and purity have been coloured for values above the average for ease of visualization. (b) Somatic mutations in the axon guidance pathway genes. The mutated genes are grouped as being involved in the following signalling cascades: Ephrins, SLIT, Semaphorins and Netrins (KEGG pathway: Axon Guidance). Figure 4: Landscape of key genetic alterations in gastric cancers. ( a ) The patient samples are shown on the x -axis. On the y -axis (top to bottom panel), the coding region mutation rate, top 12 significantly mutated genes, selected COSMIC and recurrent mutated genes, recurrent copy-number alterations (gains and deletions), clinical information, presence of TpT mutational signature, clonality, ploidy and purity are provided. The number of patients with an observed alteration type or types in given in the second column in the lower panel marked as ‘#Samples’. Different mutation and genomic alteration types are shown in different colours. Additional information is added as follows. Genes in the copy-number alterations have been marked with ‘M’ if they carried a non-synonymous mutation; ‘X’ did not show overexpression of protein by immunohistochemistry; ‘?’ for ambiguous results. The rows related to clonality, ploidy and purity have been coloured for values above the average for ease of visualization. ( b ) Somatic mutations in the axon guidance pathway genes. The mutated genes are grouped as being involved in the following signalling cascades: Ephrins, SLIT, Semaphorins and Netrins (KEGG pathway: Axon Guidance). Full size image The pathway analysis of recurrent mutations in the present study highlights cell adhesion, axon guidance and TGFB pathways ( Table 1 ). We observe that the axon guidance pathway (ephrins, netrins, semaphorins and slits) was mutated in 59% ( N =29) of the GC tumours. Frequent and exclusive mutations were grouped into the Ephrins and SLIT/ROBO pathway genes [30] , [31] ( Fig. 4b ). Table 1 Significantly mutated pathways in gastric cancer. Full size table Epstein–Barr virus-associated GC Four cancers (T07, T14, T26 and T63) were Epstein–Barr virus (EBV) positive by EBV-encoded small ribonucleic acid in situ hybridization. All four cancers were in males with diffuse-type GCs. Two modes of infection have been described, that is, chromosomal integration or episomal presence [32] . We investigated the possibility of EBV viral DNA fusion by checking the sequencing reads from all samples against 3,984 viral genomes [33] using two techniques (See methods). The EBV-positive samples were shown to have high coverage (depth in hundreds) and breadth (≥80%) for both EBV-1 and EBV-2 (See Methods and Supplementary Data 12 ). Sample T50 had very low coverage (depth in tens) of HHV-6B and following in situ hybridization testing was negative. Only one PBMC DNA sample (B07 corresponding to Tumour T07) showed minor hints of EBV infection with very low coverage depth and breadth (0.6X/38% for EBV-1, 0.4X/24% for EBV-2). All other samples were negative (coverage ≪ 0.02X and breadth ≪ 1%) for both EBV-1 and EBV-2. Several potential integration sites were identified via read pairs mapped to both human and EBV genomes but could not be validated via Sanger sequencing. Mitochondrial DNA mutations in GC Somatic mitochondrial DNA (mtDNA) mutations have been observed in cancers. Protein coding regions of mtDNA include NADH dehydrogenase (complex I), cytochrome b (complex III), cytochrome c oxidase (complex IV) and ATP synthase (complex IV). In this study, we observed 16 non-synonymous somatic mtDNA mutations in 13 GC samples ( Supplementary Data 13 ). Non-protein coding sequence regions of mtDNA include 22 tRNAs, 2 rRNAs and the displacement loop (D-loop) control region. We found three somatic mutations in mt-rRNA and four somatic mutations in mt-tRNA-related regions. Only one of the 49 GCs had a mutation in the D-loop region, which has previously been reported to be a hotspot for mutations in human GC [34] , [35] . On the basis of known polymorphisms in the human mtDNA sequence derived from >2,700 healthy individuals, we identified 24 mtDNA mutations, which have not been reported as polymorphisms [36] . The functional and clinical significances of these mutations need to be elucidated in the near future. In this study, we identified genomic alterations driving tumorigenesis, mutational signatures and clonality underlying MSS GCs spanning both intestinal and diffuse subtypes. The mutational signatures identified here divided the diffuse subtype into one with infrequent genetic changes/low clonality and another with relatively higher clonality and mutations impacting TpT dinucleotides. Overall, the diffuse-type GCs showed significantly lower clonality and smaller numbers of somatic variants compared with the intestinal-type GC. Structural analysis revealed predominantly mutually exclusive gains in receptor tyrosine kinases in a TP53 -mutant background as well as novel fusion genes. On a genetic level, TP53 was the most frequent mutation; however, the mutation patterns of TP53 in the same tumour are different and intratumoral heterogeneity exists in TP53 -inactivation mechanism. From the perspective of functionality, this should render this gene functionally ineffective in almost all cancer cells harbouring mutations of TP53. We observed significantly mutated genes in TP53 , ARID1A , TGFBR2, CDH1, SYNE1 and TMPRS S2. In recently published large-scale genomic studies on diffuse-type GCs, the prevalence of RHOA mutations varied high from 0 to 25.3% (refs 5 , 6 , 7 , 8 ). In this study with 31 diffuse-type GCs, we observed RHOA mutations in 6.5% of cases, which is lesser than GCs in Japanese patients [6] , but similar to patients in Hong Kong [8] or international consortium [5] . In addition, we discovered frequent and exclusive mutations in Ephrins and SLIT/ROBO signalling pathway genes, suggesting driver pathways in GCs. Many axon guidance molecules regulate cell migration and apoptosis in tumour [37] . Furthermore, frequent and diverse somatic aberrations in SLIT/ROBO signalling pathway have been reported in ~20% of pancreatic adenocarcinomas [38] . Knockdown of SLIT2 promotes growth and motility in GC cells via activation of AKT / CTNNB1 (β-catenin), suggesting tumour suppressor role [39] . On the basis of these findings, the Ephrins and SLIT/ROBO signalling pathways may be involved in the development of GC and could be a therapeutic target. With regards to the histological classification, we saw some remarkable differences between the intestinal and diffuse subtypes of GC. Intestinal-type tumours were more clonal with higher ploidy, suggesting that most mutations likely to occur before genome duplication event in the intestinal-type GC. TP53 -mutant group coincided with the intestinal-type GC and frequently associated with gene amplifications of receptor tyrosine kinases, cell signalling and cell cycle-related genes. This is similar to the copy-number change driven tumours (termed C-class; described in the TCGA pancancer analysis [27] ) with a strong enrichment of TP53 mutation co-occurring in this category of cancers. On the rational treatment front, these patients may have additional targeted treatment options (besides Herceptin for ERBB2 ) for inhibitors of EGFR, MET or FGFR2 for corresponding gene amplifications, CDK2 Inhibitors for CyclinE -amplified cancers and MEK inhibitors for KRAS -amplified GCs. The diffuse-type GCs tend to be more diploid, displayed lower clonality and smaller numbers of somatic alterations compared with intestinal-type GCs. A further subset of diffuse-type GCs predominantly lacked the TpT mutational signature and had very few genomic alterations, corresponding to ‘genomically stable’ tumours [5] . EBV pathogenesis and its integration into human chromosomes is still an open question. Cancers associated with EBV infection include Burkitt lymphoma, nasopharyngeal carcinoma and Hodgkin lymphoma through infection of B lymphocytes or epithelial cells. Both chromosomal integration and episomal presence have been described [32] . In our GC cases, we didn’t see any supporting evidence for EBV genome integration, suggesting that EBV may exist as an episome in the gastric tumour cells or integration exists in a small fraction of GC cells. In summary, our data provide an enhanced roadmap for the understanding of gastric adenocarcinoma with implications for future research and therapeutics in this area. GC samples Samples from 49 patients diagnosed with GC at Samsung Medical Centre, Seoul, South Korea from 2004–2007 (IRB No. 2010-12-088; patients provided their informed consent for use of samples for research) were collected and frozen at −80 °C until use. The Samsung Medical Center Institutional Review Board (IRB) approved the study protocol. Matched PBMC were also collected from all patients. No patients had undergone previous chemotherapy or radiation treatment. An expert gastrointestinal pathologist (K.M.K.) reviewed haematoxylin and eosin-stained slides to select cases with an estimated carcinoma content of >60%. In all patients, the pathologic diagnosis, histologic type by Lauren, depth of invasion and lymph node metastasis were re-evaluated. To exclude cases with MSI-high, we performed MLH1 IHC using the clone ES05 MLH1 antibody (1:100 dilution, Novocastra, UK) in formalin-fixed paraffin-embedded (FFPE) tissue sections. To assess the EBV infection status, we performed EBV-encoded small ribonucleic acid in situ hybridization. To assess the status of Helicobacter pylori infection, we evaluated previous gastric biopsy samples. Whole-genome sequencing DNA was extracted from the tumour and PBMC using the QIAamp DNA Mini Kit according to the manufacturer’s protocol (QIAGEN, Valencia, CA). DNA from both tumour and PBMC was sequenced using unchained combinatorial probe anchor ligation chemistry on arrays of self-assembling DNA nanoballs at Complete Genomics (Mountain View, CA, USA) [10] . Raw reads were aligned to human reference genome build 37.2 (National Center for Biotechnology Information (NCBI)) using Complete Genomics Analysis Pipeline v2.0. The median genome coverage was 105X for the tumours and 91X for the control. The gross mapping yields were 301.37 Gb for the tumours and 260.23 Gb for the control samples. An overview of the data delivered by the CGI pipeline is provided at http://media.completegenomics.com/documents/Overview_Data_Delivered.pdf . The corresponding data file formats (Cancer pipeline version 2 was utilized for this project) have been described in detail at the following weblink http://media.completegenomics.com/documents/DataFileFormats+Cancer+Pipeline+2.0.pdf. Hierarchical cluster The average linkage clustering with cosine distance was used for generating hierarchical cluster using Spotfire ( http://spotfire.tibco.com ). The SNV counts were converted to fractions to avoid co-clustering of samples with high single-nucleotide variant counts. Statistical tests Statistical comparison between intestinal and diffuse histologic subtypes of GC was performed via a T -test. Somatic small variation Single-nucleotide variants and small insertions and deletions were called for each sample using the calldiff method in CGA Tools v1.5 ( http://cgatools.sourceforge.net ). In brief, likelihood scores are provided for variants called in comparison with the human genome under a diploid (normal sample) or non-diploid (tumour sample) assumption. The variant and reference calls in the tumour and matched control samples are compared, with each somatic event detected by the analysis pipeline being assigned to a ‘somaticCategory’ such as SNP, insertion, deletion or block substitution. Each such event is assigned a ‘somaticScore’ reflecting the likelihood of it being true, and those events with a somaticScore of ≥10 are called SQHIGH. Three additional filtering steps were applied to boost the confidence in the read support for a called somatic variant: (1) one-side Fisher’s exact test ( P ≪ 0.05) to compare the proportion of reads supporting the somatic variant between tumour and matched PBMC samples; (2) the number of reads supporting the somatic variant in the matched PBMC should be ≤9 and (3) polymorphism filtering, in which the variants annotated as germline were removed. The filtering led to an ~20% average removal of ‘SQHIGH’ variants per tumour. Somatic mutations in mitochondrial DNA (mtDNA) were initially undetectable using CGA tools v1.5. However, based on the number of reads supporting alternative alleles and reference alleles in the tumour and matched normal samples, tumour-specific variation (that is, somatic mutations) clearly exists in the mtDNA. We used the above filters as a way to detect somatic mutations in mtDNA: (1) one-side Fisher’s exact test ( P ≪ 0.05) to select variations with a significantly higher proportion of reads supporting the somatic variant in the tumour sample; (2) the total reads supporting the somatic variant should be ≤9 in the matched normal sample; and (3) polymorphism filtering, in which removing the annotated germline variation, identified as a variant having at least three allele counts observed in a database of common polymorphisms of mtDNA annotated from 2,704 individuals ( http://www.mtdb.igp.uu.se ). The variants detected were annotated against public variant databases including 1,000 genomes (phase1 ver. 3 2010/11/23 release, http://www.1000genomes.org ), HapMap release 3.3 ( http://hapmap.ncbi.nlm.nih.gov ), NHLBI ESP Exome Variant Server (EVS) ( http://evs.gs.washington . edu/EVS), dbSNP ver. 137 ( http://www.ncbi.nlm.nih.gov/SNP ) and Complete Genomics 69 public genome ( http://www.completegenomics.com/public-data/69-Genomes ). A variant was labelled as germline if at least three allele counts were observed in the 1,000 genomes, EVS, HapMap or Complete Genomics 69 genome databases or were annotated as G5 in dbSNP (>5% minor allele frequency in more than one population). A variant was annotated as a somatic change based on COSMIC v61 ( http://cancer.sanger.ac.uk/cancergenome/projects/cosmic ). Furthermore, Snpeff v 2.1 ( http://snpeff.sourceforge.net ) was used to annotate functional changes in the WGS data. Validation of somatic mutations by targeted resequencing Recurrent genes were selected using the WGS data, and target capture oligomers were acquired from Agilent. In all, 32 of the 49 samples had sufficient DNA quantity (>1 μg) and quality to conduct the library preparation step; only one sample was omitted from further analysis. Sequencing was performed on Illumina Hiseq 2000, with an expected depth of 80X. The alignment was performed using BWA-mem v0.7.4 using the default parameters and GRCH37 as the reference genome. Variants were called by three callers: (a) samtools mpileup v0.1.19, http://samtools.sourceforge.net/ ; (b) freebayes v0.9.10, https://github.com/ekg/freebayes and c) GATK lite v2.3, http://www.broadinstitute.org/gatk /download. Variants called by at least one caller were used for both normal and tumour samples. The minimal mapping and base quality phred-like score used was Q13, and the minimum variant read support was at least three. Any tumour variants found in the paired normal samples were removed, and a cutoff of Q10 for the genotype quality score was applied. Variants found in ≥2 normal samples in this data set and likely germline variants with at least three allele counts reported in the 1,000 Genomes, EVS, HapMap and Complete Genomics 69 genome databases or annotated as G5 in dbSNP (>5% minor allele frequency in more than one population) were removed from the somatic variant list. The web locations for the data sources are listed in the section entitled ‘somatic small variation’. Significantly mutated genes We used the method previously published [16] to identify significantly mutated genes, that is, genes for which the non-silent mutation rate is significantly higher than the background mutation rate. In brief, this method incorporates information such as the functional impact of mutations on the protein products, variation in the background mutation rate among tumours and redundancy of the genetic code to provide significance. The P -value was corrected using multiple hypothesis correction with the Benjamini-Hochberg method. We also included three genes, that is, PIK3CA, APC and CTNNB1 with mutations that were reported in at least 20 tumour samples in the COSMIC v61 database. We also manually checked for spuriously significant genes [15] such as TTN , MUC16 or belonging to olfactory receptors, Cub and Sushi multi domin proteins ( CSMD ), ryanodine receptors. Among those genes, only CSMD1 and CSMD3 were present and marked out as potentially spurious ( Supplementary Data 6 ). Pathway analysis The recurrently mutated genes present in at least two samples ( N =384) were submitted to pathway enrichment analysis using DAVID v6.7 (ref. 40 ) ( http://david.abcc.ncifcrf.gov/ ). We used the KEGG, Biocarta and REACTOME pathways. The significance of enrichment was estimated using a modified Fisher exact test (as implemented at http://david.abcc.ncifcrf.gov/) and was corrected using multiple hypothesis correction with the Benjamini-Hochberg method. To address the impact of inputting different gene sets, we also submitted the list of all the genes ( N =2,553) bearing somatic non-synonymous mutations. The most significant pathways were similar across the various gene lists (data not shown). Clonality analysis To estimate the tumour sample heterogeneity, we assessed tumour purity and ploidy using ASCAT v2.1 (ref. 24 ) with γ =1 allowing ploidy to range from 1.2 to 8.0 for each tumour sample. Input files to ASCAT comprised a B-allele frequency: estimated at known polymorphic sites (based on the definition of germline variation, see section ‘somatic small variation’—variation annotation) as ratio of reads supporting the polymorphic allele in tumour sample to the total number of reads. b Relative coverage at the above polymorphic site taken from CGI file cnvDetailsDiploidBeta: estimated as the ratio of total number of reads mapping to +/− 1 kb adjacent to the polymorphic site after normalization and GC bias correction as described in online CGI documentation at http://media.completegenomics.com/documents/DataFileFormats+Cancer+Pipeline+2.0.pdf . Use of a smaller window segment size was done for allowing greater precision to estimate the relative copy number at each locus. We were unable to resolve the tumour purity and ploidy for four (T09, T49, T57 and T63) samples owing to their low number of genomic aberrations (low number of copy-number related changes). So, further manual inspection was conducted based on the solution space generated by ASCAT for each sample, and then purity and ploidy were estimated for all 49 samples. The mCN, tumour cell total copy number (tTCN) and tMAF were computed for each somatic variant in a sample, using the purity and ploidy estimates using the following equations. To distinguish between clonal and subclonal mutations, we focused on the mCN and tTCN. In the case of a clonal mutation, the mCN was expected to be close to or >1 and we used a cutoff of mCN≥0.95 to classify a mutation as clonal and subclonal otherwise. Overall, mCN, tTCN and tMAF can be utilized to infer if the mutation is clonal or not as follows. mCN≥0.95: clonal mutation, that is, present in almost all tumour cells mCN ≪ 0.95: Subclonal mutation, that is, present in a subset of tumour cells mCN ≪ 0.95 and tMAF≥0.95: special case termed subclonal-del. Likely, explanation is that heterogeneity exists through two mechanisms, that is, mutation with a copy loss in some cells along with homozygous loss in other cancer cells. Somatic structural variants Somatic structural variants in the tumour samples were identified through junctions generated from read pairs, and the junctions were grouped and resolved to identify meaningful somatic events. CGI analysis pipeline reported junctions for each sample. A junction was called by first clustering discordant mate-pair reads with similar positions and orientations, followed by local de novo assembly. Somatic junctions in the tumour samples were generated using the ‘junctiondiff’ method in CGA Tools v1.5 by evaluating those junctions found in the tumour but not in the corresponding normal tissue sample. Somatic events were called using the ‘junctions2events’ method in CGA Tools v1.5 ( http://cgatools.sourceforge.net/docs/1.5.0/ ) by analysing the identified somatic junctions, with the original junctions in the tumour sample serving as the background. The categorization and brief description from the documentation is listed here as a quick reference. Complex event involves multiple junctions and does not fit the pattern of any simple event type Deletion: deletion of the sequence Tandem duplication: tandem duplication of the origin sequence Probable inversion: inversion of the origin sequence that is confirmed from one side of the inversion only Inversion: inversion of the origin sequence replacing the sequence, confirmed from both sides Distal duplication: copy of the origin sequence into new genomic location Distal duplication by mobile element: copy of the origin sequence caused by a known active mobile element Interchromosomal: isolated junction between different chromosomes; Post-filtering was conducted on the somatic events to remove false positives by requiring at least one supporting somatic junction to have at least five mate-pair reads and a baseline frequency of ≪ 0.05. The baseline frequency of a junction defined the presence of the junction in Complete Genomics’ Diversity Panel of unrelated genomics (52 peripheral blood samples, ftp://ftp2.completegenomics.com/Baseline_Genome_set/SVBaseline ). Gene fusion candidates were reported from somatic events that linked unrelated gene regions in the genome together with identified breakpoint genomic coordinates. Genes were defined based on the annotation of protein coding regions from CCDS ( http://www.ncbi.nlm.gov/CCDS ). Gene fusion partners were examined for strand and orientation consistency and annotated for in-frame fusions. Fusion gene candidates were validated by performing RT-PCR across the fusion breakpoints followed by direct Sanger sequencing confirmation. Total mRNAs were obtained from FFPE tissue samples using an RNeasy FFPE kit (Qiagen). The RNA concentration was measured by fluorescence using a Quant-iT RNA Assay Kit (Invitrogen, Eugene, OR, USA) and RNA was reverse transcribed using a High Capacity cDNA Reverse Transcription Kit (Applied Biosystems). The RT-PCR products were amplified and then confirmed by sequencing using an ABI Prism 3130 × l DNA Sequencer (Applied Biosystems). GAPDH was used as an internal reference gene. The fusion junction sequences, PCR conditions and primer sequences were forward (F) 5′-GAGGCGGAGAAACTGACGAA-3′ and reverse (R) 5′-GCAGTTTGTCTTCATCATCTGAA-3′ for ACBD5-ZEB1 , F 5′-AAGAGTGATGGGAAGAAGTCTCTG-3′ and R 5′-GTGGAAACTTGACTGCACCG-3′ for WDR52-TGFBR2 ; F 5′-GCCGACGAGCCTACTTCAAG-3′ and R 5′-TAAGTCAACGCGCTGCAAAG-3′ for SOBP-MET , and F 5′-TGGACTCCAAAGAGCTAACTTT-3′ and R 5′-ACCTTTAACTGCTTCAGGGTCA-3′ for LACE1-MET . Somatic copy-number variations The somatic copy-number change at the gene level was summarized from the relative coverage (relCov) and further filtered by the somatic structural event information for the tumour samples. A conservative approach was taken to identify genes with copy gains or losses. The genome was segmented into 100-kb windows, with coverage at each position computed and corrected for GC bias. The average coverage for each segment was normalized to the Complete Genomics Baseline Genome Set (52 blood samples, ftp://ftp2.completegenomics.com/Baseline_Genome_set/SVBaseline ). The relative coverage (average coverage/sample median coverage) was reported from Complete Genomics’ analysis pipeline. Genes with relCov ≥4 were marked as copy gains unless a whole-gene deletion event (with no duplication detected) was reported for the gene. Borderline cases with relCov ≥1.5 and ≪ 4 required additional supporting evidence of duplication events. Similarly, genes with relCov ≤0.3 were marked as copy losses unless a whole-gene duplication event (with no deletion detected) was reported. Cases with relCov >0.3 and ≤0.6 required additional supporting evidence of a deletion event. In many cases, there was little or no change in the relCov (>0.6 and ≪ 1.5) at the gene level when examining the coverage; however, partial deletions of a gene (including at least 1 exon) were reported as somatic events. Validation of gene amplification IHC and FISH were performed in FFPE tissue sections for ERBB2 (v-erb-b2 avian erythroblastic leukaemia viral oncogene homologue 2), MET ( HGFR , hepatocyte growth factor receptor) and EGFR (epidermal-growth factor receptor) to confirm the amplification of genes identified by WGS analysis. For ERBB2 , we used the PATHWAY HER2 (4B5) rabbit monoclonal antibody (Ventana Medical Systems, no dilution required). ERBB2 FISH was done using dual-colour DNA-specific probes from PathVysion (Abbott/Vysis: LSI HER2 SpectrumOrange and CEP17 SpectrumGreen). Hybridization signals were counted in 20 nuclei per sample under a fluorescence microscope (Zeiss Axioskop; Zeiss, Germany) using recommended filter sets. In all cases, ERBB2 signal was normalized to the centromere 17 signal. ERBB2 was considered amplified when ERBB2 /CEP17 was >2.0. For MET , we used the CONFIRM anti-total MET (SP44) rabbit monoclonal primary antibody (Ventana Medical Systems, No dilution required) and MET /CEN7q FISH Probe (Abnova, Walnut, CA). For EGFR , we used the anti-NCL-L-EGFR-384 mouse monoclonal primary antibody (Novocastra, UK; 1:100 dilution). For IHC, we used Ventana BenchMark XT automated slide processing system according to the manufacturer’s protocol. In brief, 4-μm tissue sections were deparaffinized and rehydrated, and antigens were retrieved for 40 min in a citrate buffer (pH 6.1) at 95 °C. DAB was used as the chromogen, and the sections were counterstained with haematoxylin. EBV-related sequencing read detection The ‘ cgmap ’ module of Real-Time Genomics’ RTG Investigator version 2.3.2 ( http://www.realtimegenomics.com/ ) was used to map the reads generated by CGI to a collection of 3,984 viral genomes, downloaded from NCBI ( ftp://ftp.ncbi.nlm.nih.gov/genomes/Viruses/ ; retrieved on 20 June, 2012). On the basis of the mapped reads, the ‘ species ’ module of the RTG Investigator was used to calculate the species genome coverage depth (average number of reads at any given viral genomic locus) and breadth (fraction of the viral genome spanned by mated reads). Samples showing the presence of at least one virus with coverage of ≥25% of the viral genome and ≥0.5X depth are listed in Supplementary Data 13 . A second, independent mapping pipeline was used to map the same set of reads as an in silico validation of the previous results using cgmap module of RTG Investigator. All 70-bp CGI reads that did not map to the human genome by CGI pipeline were collected, separated into two 35-bp reads (read1 and read2), truncated to 20 bp to minimize gaps and separately aligned to one viral genome at a time using BWA (SAMtools, http://samtools.sourceforge.net ). The SAMtools ‘ merge ’ function was used to create mated pairs using mapped read1 and read2. Mated pairs with a distance outside of the 200 to 800 bp range (corresponding to the insert size distribution) were removed from the analysis. The results from this method (see Supplementary Data 12 ) showed high concordance with the results of the method described above using the Real-Time Genomics’ RTG Investigator version 2.3.2. Accession codes: Gastric cancer sequencing data have been deposited in the European Nucleotide Archive under the accession code PRJEB4954 ( http://www.ebi.ac.uk/ena/data/view/PRJEB495 ). How to cite this article: Wong, S. S. et al. Genomic landscape and genetic heterogeneity in gastric adenocarcinoma revealed by whole-genome sequencing. Nat. Commun. 5:5477 doi: 10.1038/ncomms6477 (2014).